Near room-temperature multiferroic materials with tunable ferromagnetic and electrical properties The quest for multiferroic materials with ferroelectric and ferromagnetic properties at room temperature continues to be fuelled by the promise of novel devices. Moreover, being able to tune the electrical polarization and the paramagnetic-to-ferromagnetic transition temperature constitutes another current research direction of fundamental and technological importance. Here we report on the first-principles-based prediction of a specific class of materials—namely, R 2 NiMnO 6 /La 2 NiMnO 6 superlattices where R is a rare-earth ion—that exhibit an electrical polarization and strong ferromagnetic order near room temperature, and whose electrical and ferromagnetic properties can be tuned by means of chemical pressure and/or epitaxial strain. Analysis of the first-principles results naturally explains the origins of these highly desired features. The search for multiferroic materials combining electric and magnetic behaviours in a single phase has attracted a lot of attention from the perspective of designing new devices [1] , [2] , [3] , [4] , [5] , [6] , [7] and deepening our knowledge of materials and electromagnetism. One particularly important current research direction aims at the discovery of materials that possess electrical polarization and are ferromagnetic at room temperature. Strikingly, it appears that these two desired features rarely coexist [4] , [6] , [8] , [9] . For instance, Bi 2 MnReO 6 and Bi 2 NiReO 6 have been predicted to exhibit an electrical polarization at room temperature, but both the Re and Ni/Mn sublattices adopt an antiferromagnetic order, therefore yielding a ‘ferrimagnetic’ rather than ferromagnetic overall ordering near 300 K (ref. 4 ). Similarly, ferrimagnetism (or weak magnetization) instead of ferromagnetism occurs in other compounds possessing a room-temperature electrical polarization, and that is the case for GaFeO 3 (ref. 6 ), hexagonal LuFeO 3 epitaxial thin films [7] and the solid solutions formed by mixing lead zirconium titanate and lead iron tantalite perovskites [10] . In other words, systems exhibiting both a significant electrical polarization and a strong magnetization near room temperature are very scarce (as also consistent with refs 11 , 12 ). On the other hand, double perovskite Bi 2 NiMnO 6 has been recently synthesized and found to be ferroelectric below 485 K and ferromagnetic below 140 K (ref. 13 ). While this latter ordering occurs below room temperature, and therefore makes Bi 2 NiMnO 6 useless for practical applications, Azuma et al. [13] have been critical in pointing out the possibility of investigating double perovskites for the search of ferromagnets having a polarization near 300 K. Double perovskite oxides R 2 NiMnO 6 (where R is a rare-earth element) [14] are thus attractive, especially since La 2 NiMnO 6 has a ferromagnetic Curie temperature T cm ~287 K and T cm is nearly linearly dependent on (and thus tunable with) the radius of the rare-earth ion in R 2 NiMnO 6 (ref. 14 ). Unfortunately, one shortcoming of the R 2 NiMnO 6 systems is that they are ‘not’ ferroelectric but rather possess antipolar displacements resulting [15] from their oxygen octahedral tilting pattern ( a − a − c + in Glazer’s notation [16] ). Nevertheless, the possibility of inducing a spontaneous electrical polarization at room temperature in R 2 NiMnO 6 -based double perovskite oxides may exist, for example, by mixing them with La 2 NiMnO 6 compounds to form short-period (001)-oriented R 2 NiMnO 6 /La 2 NiMnO 6 superlattices. As a matter of fact, recent studies [2] , [17] have shown that (001)-oriented (ABO 3 ) 1 /(A′BO 3 ) 1 superlattices can exhibit an electrical polarization if both ABO 3 and A′BO 3 materials adopt an a − a − c + tilting pattern, because of the mechanism called hybrid improper ferroelectricity [17] . It is therefore legitimate to wonder whether (001) R 2 NiMnO 6 /La 2 NiMnO 6 superlattices can be ferromagnetic and have an electrical polarization near room temperature. Here we report that such features can indeed be realized in these systems. Moreover, we show that their electrical polarization and magnetic Curie temperature can be tuned (and thus adjusted to desired values) by varying the chemical pressure (that is, the size of the rare-earth ion) and/or the epitaxial strain imposed by the substrates on which the R 2 NiMnO 6 /La 2 NiMnO 6 superlattice films can be grown. Finally, this study also allows us to better understand the mechanism of hybrid improper ferroelectricity, by providing the atomistic energy and interactions that are responsible for it in R 2 NiMnO 6 /La 2 NiMnO 6 systems. Structure and magnetic ordering in La 2 NiMnO 6 As detailed in the Methods section, first-principles calculations are performed on La 2 NiMnO 6 systems and on R 2 NiMnO 6 /La 2 NiMnO 6 superlattices for which the Ni atoms only have Mn atoms as first-nearest neighbours of the B-sublattice and vice versa . Let us first compare our predicted lattice parameters and magnetic moments of bulk La 2 NiMnO 6 , in its P2 1 / n ground state, to experimental data, in order to check the accuracy of our approach. Ferromagnetic order of Ni and Mn ions is assumed here. The a , b and c lattice vectors in the 20-atom P2 1 / n unit cell of La 2 NiMnO 6 are along the pseudo-cubic [110], [-110] and [001] directions, respectively, and their magnitudes are calculated to be 5.466, 5.425 and 7.676 Å, respectively. They therefore agree rather well (namely, within 0.73%) with the results measured at 3.5 K (ref. 18 ), which are 5.506, 5.456 and 7.732 Å, respectively. Our computed magnetic moments for Ni 2+ and Mn 4+ are 1.54 and 3.13 μ B , respectively. This is in reasonable agreement with both experimental (1.9 μ B for Ni 2+ and 3.0 μ B for Mn 4+ ) [18] and previous first-principles (1.43 μ B for Ni 2+ and 3.0 μ B for Mn 4+ ) [19] results. Ferroelectric ordering in the superlattices We initially build the R 2 NiMnO 6 /La 2 NiMnO 6 superlattices by substituting La 3+ ions by R 3+ ions in every other AO (001) plane of the perovskite structure, and then relax both atomic positions and lattice vectors. Let us do such substitution by starting from the relaxed P2 1 / n ground state of La 2 NiMnO 6 (still assuming ferromagnetic order) and replacing the second LaO layer of our 20-atom periodic supercell by RO layers (see Fig. 1a ). While the R 2 NiMnO 6 and La 2 NiMnO 6 bulk compounds exhibit a paraelectric P2 1 / n ground state, the R 2 NiMnO 6 /La 2 NiMnO 6 superlattices are all found to adopt an electrical polarization (and a polar P2 1 space group) after the full structural relaxation is reached. This electrical polarization is found here to be antiparallel to the in-plane b axis. Interestingly, we also numerically found that it can lie parallel to that axis when the R ions occupy the first, rather than second, AO layer of the 20-atom cell of our R 2 NiMnO 6 /La 2 NiMnO 6 superlattices. Figure 2a further shows that the magnitude of this polarization increases on decreasing the rare-earth ionic radius, r R , therefore revealing the possibility of continuously tuning of this polarization via the so-called chemical pressure associated with the different size of the rare-earth ions [20] , [21] . 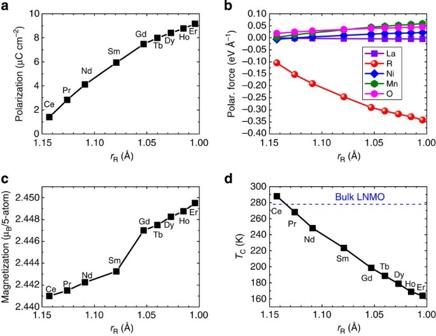Figure 2: Properties of R2NiMnO6/La2NiMnO6systems as a function of the rare-earth ionic radius. (a,c,d) The predicted electric polarization (as computed from Berry phase), magnetization (atT=0 K) and paramagnetic-to-ferromagnetic transition temperature (as calculated by Monte Carlo simulation) in the relaxed P21ground state of the superlattices, respectively. (b) The average forces (along thebdirection) on La3+, R3+, Ni2+, Mn4+and O2−ions in the unrelaxed state of the R2NiMnO6/La2NiMnO6superlattice, for which the lattice parameters and atomic coordinates are those of the paraelectric P21/nstate of La2NiMnO6and for which the R ions occupy the second AO layer ofFig. 1a. The blue horizontal dashed line indrepresents the magnetic Curie temperature of La2NiMnO6bulk. As evidenced inSupplementary Fig. 2, the error bar of the paramagnetic-to-ferromagnetic transition temperature can be estimated to be about 6 K. Moreover, an error bar of polarization can be estimated by comparing the results of the relaxed structure of the Er2NiMnO6/La2NiMnO6superlattice when usingU=3 eV andU=5 eV. It is found to be as small as 1% (which corresponds to a variation of the polarization from 9.16 to 9.26 μC cm−2). In fact, since the ionic radius of La in La 2 NiMnO 6 or R 2 NiMnO 6 /La 2 NiMnO 6 material is about 1.16 Å (ref. 22 ; La has a coordination number of eight in these compounds), Fig. 2a also shows that the in-plane electrical polarization is enhanced when the difference of ionic radius between R and La increases. Practically, the electrical polarization ranges between 1.4 μC cm −2 for the Ce 2 NiMnO 6 /La 2 NiMnO 6 system and 9.2 μC cm −2 for the Er 2 NiMnO 6 /La 2 NiMnO 6 superlattice, such values being large enough to be experimentally detected. They are also of the same order as the in-plane electrical polarization predicted to exist, via the so-called hybrid improper ferroelectricity, in the BiFeO 3 /LaFeO 3 superlattice grown on a (001)-oriented SrTiO 3 substrate [2] and in some other (ABO 3 ) 1 /(A′BO 3 ) 1 superlattices [17] combining two pure ABO 3 and A′BO 3 materials that adopt the a − a − c + tilting pattern and are paraelectric. 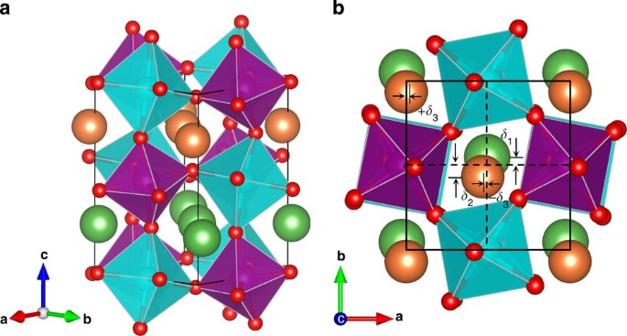(Note that a and c in this notation of the tilting pattern refer to rotations around the pseudo-cubic <001> axes.) Figure 1: P21ground state of the studied R2NiMnO6/La2NiMnO6superlattices. (a) Representation in three dimensions. (b) Representation in the (a,b) plane. The La3+, R3+, Ni2+, Mn4+and O2−ions are displayed as green, orange, cyan, purple and red spheres, respectively. The NiO6and MnO6octahedra are displayed using cyan and purple octahedra, respectively. The largest magnitude of the antipolar displacement (δ2) of the R3+ions with respect to those (δ1) of the La3+ions along thebaxis is schematized here to emphasize that this inhomogeneity is the microscopic reason for the creation of the electrical polarization. The antipolar displacements along theaaxis of the R ions within the RO plane (denoted as +δ3and −δ3) are also shown. As examples,δ1,δ2andδ3are equal to 0.048, 0.070 and 0.017, respectively, in lattice constant units in Er2NiMnO6/La2NiMnO6(and 0.024, 0.027 and 0.006, respectively, in Ce2NiMnO6/La2NiMnO6). Figure 1: P2 1 ground state of the studied R 2 NiMnO 6 /La 2 NiMnO 6 superlattices. ( a ) Representation in three dimensions. ( b ) Representation in the (a,b) plane. The La 3+ , R 3+ , Ni 2+ , Mn 4+ and O 2− ions are displayed as green, orange, cyan, purple and red spheres, respectively. The NiO 6 and MnO 6 octahedra are displayed using cyan and purple octahedra, respectively. The largest magnitude of the antipolar displacement ( δ 2 ) of the R 3+ ions with respect to those ( δ 1 ) of the La 3+ ions along the b axis is schematized here to emphasize that this inhomogeneity is the microscopic reason for the creation of the electrical polarization. The antipolar displacements along the a axis of the R ions within the RO plane (denoted as + δ 3 and − δ 3 ) are also shown. As examples, δ 1 , δ 2 and δ 3 are equal to 0.048, 0.070 and 0.017, respectively, in lattice constant units in Er 2 NiMnO 6 /La 2 NiMnO 6 (and 0.024, 0.027 and 0.006, respectively, in Ce 2 NiMnO 6 /La 2 NiMnO 6 ). Full size image Figure 2: Properties of R 2 NiMnO 6 /La 2 NiMnO 6 systems as a function of the rare-earth ionic radius. ( a , c , d ) The predicted electric polarization (as computed from Berry phase), magnetization (at T =0 K) and paramagnetic-to-ferromagnetic transition temperature (as calculated by Monte Carlo simulation) in the relaxed P2 1 ground state of the superlattices, respectively. ( b ) The average forces (along the b direction) on La 3+ , R 3+ , Ni 2+ , Mn 4+ and O 2− ions in the unrelaxed state of the R 2 NiMnO 6 /La 2 NiMnO 6 superlattice, for which the lattice parameters and atomic coordinates are those of the paraelectric P2 1 / n state of La 2 NiMnO 6 and for which the R ions occupy the second AO layer of Fig. 1a . The blue horizontal dashed line in d represents the magnetic Curie temperature of La 2 NiMnO 6 bulk. As evidenced in Supplementary Fig. 2 , the error bar of the paramagnetic-to-ferromagnetic transition temperature can be estimated to be about 6 K. Moreover, an error bar of polarization can be estimated by comparing the results of the relaxed structure of the Er 2 NiMnO 6 /La 2 NiMnO 6 superlattice when using U =3 eV and U =5 eV. It is found to be as small as 1% (which corresponds to a variation of the polarization from 9.16 to 9.26 μC cm −2 ). Full size image Interestingly, our superlattices also possess a similar tilting pattern, with antiphase tilting of the NiO 6 and MnO 6 octahedra in the (a,b) plane as well as in-phase tilting about the out-of-plane c direction. Let us therefore determine whether the mechanism of hybrid improper ferroelectricity, that technically relies on an energy of the form λQ 1 Q 2 P based on symmetry arguments (where λ is a constant, Q 1 and Q 2 are in-plane antiphase and out-of-plane in-phase tilting modes, respectively, and P is the in-plane polarization), also applies to our investigated systems. If it does apply, we also wish to provide a microscopic understanding for the formation of the electrical polarization in our systems. For that, it is important to first recall that Bellaiche and Íñiguez [15] demonstrated, via the introduction of specific atomistic interactions giving rise to the energy that was denoted Δ E 1 , that any a − a − c + tilting pattern in any perovskite material should also generate antipolar motions of the A atoms that are parallel to the b direction in one (001) AO plane and then antiparallel to the b axis in the next (001) AO plane. Such antipolar displacements of the La ions are indeed numerically found in the relaxed P2 1 / n state of bulk La 2 NiMnO 6 . We then decided to start from this latter state of La 2 NiMnO 6 (adopting ferromagnetism), then substitute the second LaO layer by an RO layer (in our periodic 20-atom supercell) to create the R 2 NiMnO 6 /La 2 NiMnO 6 superlattice shown in Fig. 1a , but preventing any ionic relaxation from occurring after such substitution is done. The resulting average forces along the b direction for all types of ions are displayed in Fig. 2b as a function of the rare-earth ionic radius [22] . Note that there are no average forces on any kind of atom along the a and c axes and, by average force, we mean the sum of the forces on the same kind of atoms divided by the number of these forces. Three important features are revealed by this figure. First of all, the force on the R 3+ ions is the dominant one among all forces felt by ions along the b direction. Second, this force on the R 3+ ions is antiparallel to the b axis (interestingly, we further found that this force is parallel to the b direction if the R ions occupy the first AO layer). Third, the magnitude of this force increases as r R decreases. It is thus clear that the electrical polarization of the fully relaxed R 2 NiMnO 6 /La 2 NiMnO 6 superlattices shown in Fig. 2a mostly originates from the fact that the opposite antipolar motions (along the b direction) of R and La ions do not have the same magnitude, as schematized in Fig. 1b and also consistent with refs 2 , 23 . Such an inhomogeneity of antipolar motions can be understood when realizing that the Δ E 1 atomistic energy provided in ref. 15 naturally leads (because of the a − a − c + tilting pattern) to the (001) LaO layers of Fig. 1 experiencing a ‘global, macroscopic-like’ energy of the form −K 1,La ω R ω M u La where K 1,La is a positive constant, ω R and ω M are scalars characterizing the in-plane antiphase and out-of-plane in-phase tiltings, respectively [24] , and u La is the displacement of the La ions along the b axis with respect to their ideal positions. Similarly, the (001) RO layers of Fig. 1 have an associated energy of the form +K 1,R ω R ω M u R , where K 1,R is another positive constant (which is different from K 1,La because of the different chemical nature of the AO layers) and u R is the displacement of the R ions along the b direction. By summing these two different energies and introducing the polarization P=(u La +u R )/2 and an antiferroelectric vector A=(u La − u R )/2 (associated with the X-point of the five-atom cubic Brillouin zone), one obtains a total energy that can be decomposed into two novel parts, namely −(K 1,La +K 1,R )ω R ω M A and −(K 1,La −K 1,R )ω R ω M P. The former is responsible for the existence of a homogenous in-plane antiferroelectric vector in the superlattice, while the latter precisely characterizes the so-called hybrid improper ferroelectricity [17] , [23] . Note that the effective charges of La and R ions are found to be rather similar along the b axis (namely, around 4.15), with their differences typically ranging between 2% (when R=Ce) and 7% (when R=Er). One can thus directly relate polarization with ionic displacements of La and R ions, in first approximation (we numerically found that the difference in effective charges between La and R ions typically results in a change of a polarization that is five times smaller than the polarization arising from the assumption that La and R ions have the same average effective charge in the R 2 NiMnO 6 /La 2 NiMnO 6 superlattices). Note also that the fact that Fig. 2a shows that the magnitude of the polarization is enhanced when the difference in size between the R and La ions increases implies that the coefficient in front of the second aforementioned energy, namely K 1,La −K 1,R , becomes larger as the size difference between R and La ions is bigger. Interestingly, if we start again from the symmetry–invariant energy Δ E 1 provided in ref. 15 and consider the same tilting pattern as above (that is, same values of ω R and ω M ), but choose the alternate ordering of the (001) LaO and RO planes (that is, with respect to the example above, we exchange the locations of La and R atoms), one can show that the polarization-inducing energy term turns out to be −(K 1,R −K 1,La )ω R ω M P, that is, the same as above but with opposite sign. The minimization of this energy, via structural relaxation of the A atoms, implies that the polarization will then switch its direction when the R ions occupy the first (rather than the second) AO layer of the used 20-atom periodic supercell. Note that, ultimately, the phase matching between the La/R ordering and the antiphase rotations ω R determines the polarization direction. Note also that, and as demonstrated in refs 2 , 25 , the polarization of systems possessing trilinear coupling energy (as it is the case here) is switchable, which also typically leads to a switch of oxygen octahedral tiltings. It will also be interesting to determine in future studies whether this polarization switching is homogenous or (non)inhomogenous in nature (especially when defects are present in the grown sample). Finally, let us point out that, as shown in Fig. 1b , any two first-nearest neighbouring R (respectively, La) ions in any (001) AO plane move in an antiparallel manner to each other along the a axis—that is, along the in-plane direction that is perpendicular to the polarization. Such an additional displacement originates from the Δ E 2 atomistic energy of ref. 15 , which induces another antiferroelectric vector (in this case associated with the R-point of the five-atom cubic Brillouin zone) as a result of the a − a − c + tilting pattern. Such additional displacements average out to zero in any (001) AO plane, and therefore do not give rise to any component of the macroscopic spontaneous polarization along the a axis. Magnetic ordering in the superlattices Having understood the origin of the polarization in the R 2 NiMnO 6 /La 2 NiMnO 6 superlattices, it is clear that this polarization should remain non-zero at room temperature since the energy −(K 1,La −K 1,R )ω R ω M P implies that the polarization is driven by the oxygen octahedral tiltings and both the antiphase and in-phase oxygen octahedral tiltings are known to exist at ambient conditions in both La 2 NiMnO 6 and R 2 NiMnO 6 pure materials [26] . Let us now check whether these superlattices can also exhibit a significant magnetization at 300 K, which would thus make them room-temperature multiferroics. First, note that Fig. 2c shows that the computed magnetization of the R 2 NiMnO 6 /La 2 NiMnO 6 superlattices at T =0 K is large (of the order of 2.4–2.5 Bohr magneton per five atoms) for any R ion, as consistent with a strong ferromagnetism. To determine whether this magnetization can persist up to room temperature, we calculate the paramagnetic-to-ferromagnetic Curie point of R 2 NiMnO 6 /La 2 NiMnO 6 superlattices (see Fig. 2d ). We first investigate the Curie temperature of bulk R 2 NiMnO 6 and La 2 NiMnO 6 double perovskites as a function of the rare-earth ionic radius, arising from the use of different Hubbard U values (see Supplementary Fig. 1 and Supplementary Discussion ). The calculated Curie temperatures are systematically overestimated compared with the experimental values [14] . In addition, the increasing of Hubbard U enhances T C in bulk R 2 NiMnO 6 and La 2 NiMnO 6 . Thus, we multiplied the first-principles-derived exchange constants (with Hubbard U 3.0 eV for both Ni and Mn) of all the spin Hamiltonians used in this work by a factor of 0.685, which is the correction needed so that the Heisenberg Hamiltonians reproduce all the experimental paramagnetic-to-ferromagnetic transition temperatures of the different R 2 NiMnO 6 systems [14] (see Supplementary Fig. 2 and Supplementary Discussion ). The calculated Curie temperature of R 2 NiMnO 6 /La 2 NiMnO 6 superlattices decreases from ~290 to ~165 K when going from R=Ce to R=Er. As a result, the magnetic temperature of R 2 NiMnO 6 /La 2 NiMnO 6 is significantly tunable (that is, by >100 K) via the chemical pressure associated with the size of the R ions, and Ce 2 NiMnO 6 /La 2 NiMnO 6 superlattice is a specifically promising candidate for designing a near room-temperature multiferroic material. These two findings are of obvious technological importance. Please note that our calculated Curie temperature of Ce 2 NiMnO 6 /La 2 NiMnO 6 superlattice is the largest one compared with the other eight R 2 NiMnO 6 /La 2 NiMnO 6 superlattices as well as bulk La 2 NiMnO 6 . This leads us to gain more insight into La 2 NiMnO 6 and R 2 NiMnO 6 . Thus we investigate the correlation between Curie temperature of bulk R 2 NiMnO 6 perovskites and antiphase as well as in-phase tilting angles (see Supplementary Figs 3 and 4 and Supplementary Discussion ). Effects of epitaxial strain on physical properties All the aforementioned calculations concern fully relaxed R 2 NiMnO 6 /La 2 NiMnO 6 systems. However, in some cases, some lattice vectors are imposed by external conditions and thus cannot relax to their equilibrium values. This is the case for epitaxial (001) thin films, for which the in-plane lattice parameters are those of the substrate on top of which the films are grown. It is thus relevant to investigate the effect of an epitaxial misfit strain on properties of the R 2 NiMnO 6 /La 2 NiMnO 6 superlattices. For that purpose, the calculated electric polarization and Curie temperature of (001)-oriented films made of Ce 2 NiMnO 6 /La 2 NiMnO 6 , Pr 2 NiMnO 6 /La 2 NiMnO 6 , Sm 2 NiMnO 6 /La 2 NiMnO 6 , Er 2 NiMnO 6 /La 2 NiMnO 6 and La 2 NiMnO 6 , are shown in Fig. 3a,b as a function of the in-plane lattice parameter (a IP ). Our calculated results first show that the electric polarization of the investigated R 2 NiMnO 6 /La 2 NiMnO 6 superlattices is basically independent of the epitaxial strain, with the exception of Er 2 NiMnO 6 /La 2 NiMnO 6 for which the polarization slightly increases from ~9.0 to ~10.5 μC cm −2 when a IP decreases from 3.96 to 3.68 Å. This insensitivity of the polarization with strain is technologically useful since it implies that the polarization persists for a large choice of available substrates. It is also fundamentally interesting since it goes against the common knowledge that in-plane polarization of (001) films should rapidly decrease, and even disappear, when decreasing the in-plane lattice constant (that is, when the strain becomes compressive and large in magnitude) [27] , [28] , [29] . In fact, and as consistent with what was recently found for rare-earth orthochromates [20] , such a unusual and weak dependence of the in-plane polarization on the strain is due to the fact that a larger epitaxial compression tends to reduce the in-plane antiphase tilting ω R while increasing the out-of-plane in-phase tilting ω M . As a result, the product ω R ω M is largely independent of the strain, and so is the in-plane polarization that depends on this ω R ω M product via the aforementioned hybrid improper ferroelectricity mechanism. 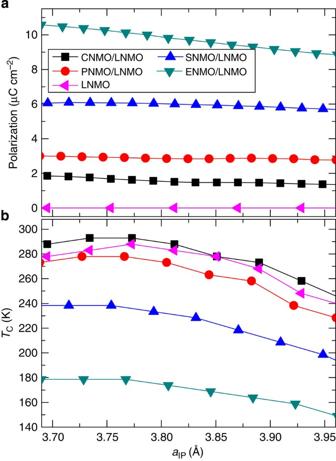Figure 3: Properties of epitaxial (001) films made of several superlattices as a function of the in-plane lattice parameter. These superlattices are Ce2NiMnO6/La2NiMnO6(CNMO/LNMO), Pr2NiMnO6/La2NiMnO6(PNMO/LNMO), Sm2NiMnO6/La2NiMnO6(SNMO/LNMO), Er2NiMnO6/La2NiMnO6(ENMO/LNMO) and La2NiMnO6(LNMO), as a function of the in-plane lattice parameter. (a) The electric polarization as computed from Berry phase. (b) The magnetic Curie temperature as calculated by Monte Carlo simulation. As indicated in the captions ofFig. 2, the error bar for the polarization is estimated to be of the order of 1% while the error bar of the paramagnetic-to-ferromagnetic transition temperature is estimated to be about 6 K. Figure 3: Properties of epitaxial (001) films made of several superlattices as a function of the in-plane lattice parameter. These superlattices are Ce 2 NiMnO 6 /La 2 NiMnO 6 (CNMO/LNMO), Pr 2 NiMnO 6 /La 2 NiMnO 6 (PNMO/LNMO), Sm 2 NiMnO 6 /La 2 NiMnO 6 (SNMO/LNMO), Er 2 NiMnO 6 /La 2 NiMnO 6 (ENMO/LNMO) and La 2 NiMnO 6 (LNMO), as a function of the in-plane lattice parameter. ( a ) The electric polarization as computed from Berry phase. ( b ) The magnetic Curie temperature as calculated by Monte Carlo simulation. As indicated in the captions of Fig. 2 , the error bar for the polarization is estimated to be of the order of 1% while the error bar of the paramagnetic-to-ferromagnetic transition temperature is estimated to be about 6 K. Full size image Moreover, Fig. 3b shows that the paramagnetic-to-ferromagnetic Curie temperature of the superlattices (and La 2 NiMnO 6 ) is rather sensitive to the epitaxial strain, as consistent with ref. 30 and magnetostriction: as a IP decreases, the Curie temperature goes up significantly at first, to eventually become weakly a IP dependent. Figure 3b therefore shows that one can also create a near room-temperature multiferroic, and tune magnetic transition temperature, by applying an appropriate epitaxial strain in the R 2 NiMnO 6 /La 2 NiMnO 6 superlattices. In particular, (001) Ce 2 NiMnO 6 /La 2 NiMnO 6 films are promising materials to exhibit magnetization and polarization above 290 K, when grown on any substrate having an in-plane lattice constant ranging between 3.70 and 3.80 Å (which corresponds to an average compressive epitaxial strain experienced by Ce 2 NiMnO 6 /La 2 NiMnO 6 films varying between −3.9% and −1.3%). We have discovered that (and understood why) (001)-oriented R 2 NiMnO 6 /La 2 NiMnO 6 superlattices can adopt an electrical polarization and be ferromagnetic essentially up to room temperature. Moreover, our first-principles calculations also reveal that the electric and magnetic properties can be tuned by chemical pressure and/or epitaxial strain in these systems. We thus hope that our predictions will soon be experimentally confirmed and used to design novel spintronic devices. Note that these predictions are for R 2 NiMnO 6 /La 2 NiMnO 6 superlattice systems that are perfectly chemically ordered, and that disordering on the A- or B-sites likely will affect physical properties. It is thus important for experimentalists to fully control atomic ordering in the grown samples in order to be able to check our predictions. We are optimistic that our proposed R 2 NiMnO 6 /La 2 NiMnO 6 superlattices will be successfully grown in a near future based on the facts that similar compounds (namely, NaRMnWO 6 and, especially, Bi 2 NiMnO 6 /La 2 NiMnO 6 superlattices) have already been synthesized [31] , [32] . Note also that polarization and magnetism are coupled in our R 2 NiMnO 6 /La 2 NiMnO 6 superlattices since polarization is typically found to be enhanced by around 3% when going from the ferromagnetic to ferrimagnetic state (for which Mn and Ni ions being nearest neighbours to each other have opposite direction of their magnetic moment as well as different magnitudes for these moments). It is also important to realize that not all possible devices using multiferroics require a strong coupling between polarization (P) and magnetization (M). For instance, one can think of a four-state memory for which +/−P and +/−M can be accessed by using electric and magnetic fields, respectively, and for which it is desired to have a weak (rather than strong) coupling between P and M [33] . We also hope that other room-temperature ferromagnetic multiferroics will be discovered following the general design principles employed here—namely: to combine two paraelectric compounds that are both ferromagnetic within a superlattice, create an electrical polarization in the resulting superlattice via the so-called hybrid improper ferroelectricity mechanism, and tune electrical and magnetic properties of the superlattice by chemical pressure or epitaxial strain. Calculation of structure and ferroelectric polarization First-principles calculations are performed on La 2 NiMnO 6 systems and on R 2 NiMnO 6 /La 2 NiMnO 6 superlattices by using the Vienna ab initio Simulation Package (VASP) within the framework of the projected augmented wave method [34] . As consistent with ref. 14 , a specific chemical ordering is assumed for all these compounds so that, within the B-sublattice, Ni atoms only have Mn atoms as first-nearest neighbours and vice versa . Practically, we investigate R=Ce, Pr, Nd, Sm, Gd, Tb, Dy, Ho and Er, and R 2 NiMnO 6 /La 2 NiMnO 6 superlattices are built from La 2 NiMnO 6 by replacing every other (001) LaO plane by a plane with RO composition (see Fig. 1 drawn by VESTA code [35] ). The generalized gradient approximation GGA+U method with the parameterization of Perdew–Burke–Ernzerh revised for solids (PBEsol) [36] is used in the present work. The effective on-site Coulomb interaction is selected to be 3 eV for both Ni 2+ and Mn 4+ ions, in line with typical choices in the literature [19] , [37] . We treat the valence electron configuration as follows: 5 s 2 5 p 6 5 d 1 6 s 2 for La, Ce, Pr, Nd, Sm; 5 p 6 5 d 1 6 s 2 for Gd, Tb, Dy, Ho, Er; 3 d 9 4 s 1 for Ni; 3 d 6 4 s 1 for Mn; and 2 s 2 2 p 4 for O. The 4 f electrons of rare-earth ions are thus kept as core electrons owing to the fact that partially filled f orbitals are usually not well described by the current density functional theory (see, for example, ref. 34 ) and the properties studied in this article can be well mimicked without explicitly treating the 4 f electrons. For instance, Supplementary Fig. 2 shows that the experimental Curie temperatures of bulks R 2 NiMnO 6 of ref. 14 can be very well reproduced without the need to incorporate 4 f electrons in the valence, which is consistent with the known facts that 4 f electrons only contribute to magnetism at very low temperature [26] . Similarly, we numerically found that the inclusion of the 4 f electrons has a relatively small effect on structural properties at 0 K, as demonstrated by the change of the a, b and c lattice parameters of Gd 2 NiMnO 6 by only 0.5%, 0.08% and 0.4%, respectively, with respect to the case when these 4 f electrons are kept in the core. We also use a plane wave energy cut-off of 500 eV and a 6 × 6 × 4 k -point mesh for Brillouin zone integrations. Structural optimizations were stopped when forces were <0.005 eV Å −1 . The space group of the different phases encountered in the present work is determined by using the FINDSYM software [38] and the electric polarization is calculated by the Berry phase approach [39] (note that the electric polarization is evaluated by choosing the P2 1 / n ground state of bulk La 2 NiMnO 6 as reference). Calculation of magnetic Curie temperature The in-plane and out-of-plane magnetic exchange constants J Ni-Mn determined from our first-principles calculations are taken as input for an effective Heisenberg Hamiltonian H =½Σ J Ni-Mn S Ni · S Mn , where we assume classical spins and take | S Ni |=| S Mn |=1 for simplicity (these exchange constants are reported in Supplementary Tables 1 and 2 ). To compute the magnetic ordering temperatures, we solve such Hamiltonians by means of Monte Carlo simulations [40] of a 20 × 20 × 20 periodically repeated simulation supercell that contains 4,000 Ni spins and 4,000 Mn spins. We use 40,000 Monte Carlo sweeps for thermalization and 60,000 additional sweeps for computing statistical averages. Finally, note that we multiplied the first-principles-derived exchange constants of all the spin Hamiltonians used in this work by a factor of 0.685, which is the correction needed so that the Heisenberg Hamiltonians reproduce all the experimental paramagnetic-to-ferromagnetic transition temperatures of the different R 2 NiMnO 6 systems reported in ref. 14 (see Supplementary Fig. 2 ). How to cite this article: Zhao, H. J. et al. Near room-temperature multiferroic materials with tunable ferromagnetic and electrical properties. Nat. Commun. 5:4021 doi: 10.1038/ncomms5021 (2014).